Novel pleiotropic risk loci for melanoma and nevus density implicate multiple biological pathways The total number of acquired melanocytic nevi on the skin is strongly correlated with melanoma risk. Here we report a meta-analysis of 11 nevus GWAS from Australia, Netherlands, UK, and USA comprising 52,506 individuals. We confirm known loci including MTAP , PLA2G6 , and IRF4 , and detect novel SNPs in KITLG and a region of 9q32. In a bivariate analysis combining the nevus results with a recent melanoma GWAS meta-analysis (12,874 cases, 23,203 controls), SNPs near GPRC5A, CYP1B1 , PPARGC1B , HDAC4 , FAM208B, DOCK8 , and SYNE2 reached global significance, and other loci, including MIR146A and OBFC1, reached a suggestive level. Overall, we conclude that most nevus genes affect melanoma risk ( KITLG an exception), while many melanoma risk loci do not alter nevus count. For example, variants in TERC and OBFC1 affect both traits, but other telomere length maintenance genes seem to affect melanoma risk only. Our findings implicate multiple pathways in nevogenesis. The incidence of cutaneous malignant melanoma (CM) has increased in populations of European descent in North America, Europe, and Australia due to long-term changes in sun exposure behavior, as well as screening [1] . The strongest CM epidemiological risk factor acting within populations of European descent is the number of cutaneous acquired melanocytic nevi, with risk increasing by 2–4% per additional nevus counted [2] . Nevi are benign melanocytic tumors usually characterized by a signature somatic BRAF mutation. Their association with CM can be direct, in that a proportion of melanomas arise within a pre-existing nevus (due to a “second hit” mutation), or indirect, where genetic or environmental risk factors for both traits are shared. Total nevus count is highly heritable (60%–90% in twins) [3] , [4] , but only a small proportion of this genetic variance is explained by loci identified so far [5] , [6] , [7] , [8] , [9] . The known nevus count loci all have pleiotropic effects on CM risk [5] , [6] , [7] , [8] , [9] , which implies both that nevus count loci are medically important and that a genetic analysis combining nevi and CM phenotypes will have increased statistical power. Here we present a new large nevus genome-wide association meta-analysis, and combine these results with those of a previously published meta-analysis of melanoma [10] . 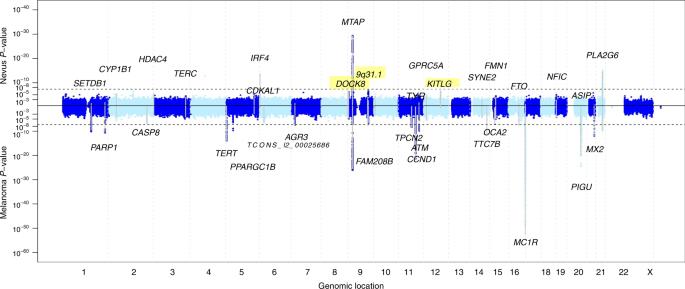Fig. 1 Miami plot of nevus count and melanoma meta-analysis.Pvalues where eitherP< 10−5. The –log10Pvalues for the nevus GWAS meta-analysis are above the central solid line and those for the melanoma GWAS meta-analysis are below that line. Novel nevus loci are highlighted Nevus GWAS meta-analysis Genome-wide single-nucleotide polymorphism (SNP) genotype data were available for a total of 52,806 individuals from 11 studies in Australia, UK, USA, and the Netherlands (Table 1 ), where nevus number had been measured by counting or ratings, by self or observer, and of the whole body or selected regions. Analyses show that these are measuring the same entity and are therefore combinable for GWAS (genome-wide association study; see Supplementary Results). The genomic inflation factors were λ = 1.41 and λ 1000 = 1.008 (Q–Q plot, Supplementary Fig. 1 ), consistent with polygenic inheritance and the total sample size. [11] Five genomic regions contained association peaks that reached genome-wide significance in the nevus count meta-analysis (Fig. 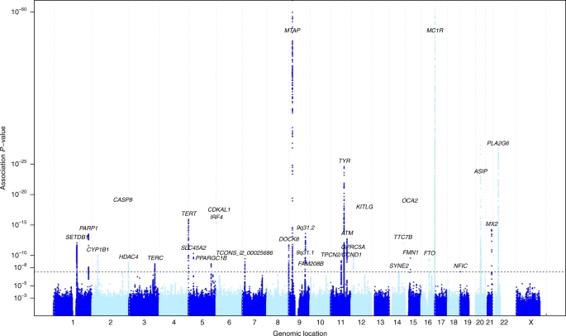Fig. 2 Manhattan plot ofPvalues from meta-analysis combining nevus and melanoma results 1 , Table 2 , Supplementary Fig. 2 ), MTAP/CDKN2A on chromosomes 9p21.3 (peak SNP, P = 2 × 10 −37 ) and 9q31.1-2 ( P = 1 × 10 −8 ), IRF4 on chromosome 6p (peak SNP, P = 4 × 10 −37 ), in KITLG in the region of the known testicular germ cell cancer risk locus ( P = 8 × 10 −9 ), rs600951 over DOCK8 on chromosome 9p24.3 ( P = 2 × 10 −8 ), and PLA2G6 on chromosome 22 ( P = 3 × 10 −18 ). We have previously detected three of these in analyses using subsets of the meta-analysis sample [5] , [10] . A SNP, rs251464, in PPARGC1B ( P = 5 × 10 −7 ), reached a suggestive level of association. We detected statistical heterogeneity in association with nevus count especially for IRF4 , MTAP , PLA2G6 , and DOCK8 (see Supplementary Tables 1 and 2 )—that for IRF4 was expected—given our original studies of this gene showing crossover G × age interaction. [10] Meta-regression including age of the current study participants confirmed the age effect in the case of IRF4 (Supplementary Table 1 ). Table 1 GWAS studies of nevus count contributing to the present meta-analysis Full size table Fig. 1 Miami plot of nevus count and melanoma meta-analysis. P values where either P < 10 −5 . The –log10 P values for the nevus GWAS meta-analysis are above the central solid line and those for the melanoma GWAS meta-analysis are below that line. Novel nevus loci are highlighted Full size image Table 2 SNPs associated with total nevus count and cutaneous melanoma (CM) in their respective meta-analyses Full size table Combining nevus and melanoma GWAS meta-analyses—Bayesian analysis We then combined these nevus meta-analysis P values with those from the melanoma meta-analysis [10] (Table 1 , Fig. 2 , Supplementary Figs 1, 2). We used simple combination of P values (weighted Stouffer method), as well as the GWAS-PW program, [12] which combines GWAS data for two related traits to investigate the causes of genetic covariation between them (see Supplementary Methods ). Specifically, it estimates Bayes factors and posterior probabilities of association (PPA) for four hypotheses: (a) a locus specifically affects melanoma only or (b) affects nevus count only; (c) a locus has pleiotropic effects on both traits; and (d) there are separate alleles at a locus independently determining each trait (colocation). Fig. 2 Manhattan plot of P values from meta-analysis combining nevus and melanoma results Full size image There were 30 regions containing SNPs that met our threshold for “interesting” (PPA > 0.5) for any of these hypotheses (Fig. 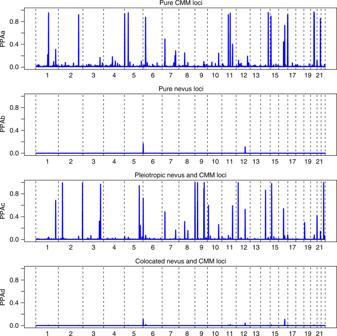Fig. 3 Results of analyses using GWAS-PW, which assign posterior probabilities (PPA) to each of ~ 1700 genomic regions that isaa pure melanoma locus,ba pure nevus locus,ca pleiotropic nevus and melanoma loci, anddthat the locus contains co-located but distinct variants for nevi and melanoma 3 , Supplementary Table 3 ). Twelve of these loci exhibited no evidence of association to nevus count, but were strongly associated with melanoma risk, one of the most extreme being MC1R . A total of 18 loci showed pleiotropic action with consistent directional and proportional effects of all SNPs on nevi and melanoma risk, the strongest being MTAP, PLA2G6 , and an intergenic region on 9q31.1 (Fig. 4a shows a bivariate regional association around GPRC5A , all loci are shown in Supplementary Figs 5 – 19 ). There were no “pure nevus” regions using the binned GWAS-PW test (hypothesis b, PPAb > 0.2), with even the region of KITLG appearing as a pleiotropic region (PPAb = 0.52, PPAc = 0.11), even though the pattern of bivariate association appears more consistent with a “nevus-only” locus (Fig. 4b ). For another five regions, support was split between the pure melanoma and pleotropic models. In the case of IRF4 , this is certainly driven by the marked between-study heterogeneity in melanoma association due to their different age distributions and latitudinal origins [13] . Fig. 3 Results of analyses using GWAS-PW, which assign posterior probabilities (PPA) to each of ~ 1700 genomic regions that is a a pure melanoma locus, b a pure nevus locus, c a pleiotropic nevus and melanoma loci, and d that the locus contains co-located but distinct variants for nevi and melanoma Full size image Fig. 4 Plot of nevus and melanoma association test P values for a the region around rs1640875 in GPRC5A (chr12:12.9 Mbp) illustrating symmetrical influence on nevus count and melanoma risk; note that neither univariate peaks achieve significance alone but in combination they do (see Table 2 , Fig. 2 ), and b the region around rs7313352 in KITLG (chr12:88.6 Mbp), a “pure” nevus locus with negligible direct effect on melanoma risk Full size image One interesting SNP (rs34466956), 2 kbp upstream from NFIC on chromosome 19p13.3 (see Fig. 5 ), achieved a combined P value of 3 × 10 −8 and a SNP-wise PPAc for pleiotropism of 0.9, even though the binned GWAS-PW assigned the region a highest PPA of 0.28. Fig. 5 UCSC Genome Browser view of region near NFIC (19p13.3). The pale blue line highlights location of rs34466956, which coincides with a narrow regulatory region as seen in in the 22 short red bars indicating open chromatin in melanocytes and skin. These align in the bottom 6 tracks with narrow yellow regions indicating results of hidden Markov models summarizing the evidence from multiple experiments for open chromatin in melanocytes. An MITF ChipSeq peak also overlies this same region (gray track, GSM1517751). NFIC is expressed in melanocytes, and a second larger MITF peak overlies intron 1 in two ChipSeq experiments viz. GSE50681_MITF, see short solid black bar, and also the tall sharp gray peak below it in GSM1517751. See Supplementary Methods for details Full size image Pleiotropy The 18 pleiotropic loci each come from multiple pathways, indicating that nevogenesis is a more complicated process than previously anticipated. Pathways already implicated include those of MTAP (purine salvage pathway, possibly a rate limiting step to cell proliferation), PLA2G6 (phospholipase A2, implicated in apoptosis), and IRF4 (melanocyte pigmentation and proliferation). Newly implicated here in nevogenesis, TERC is a strong candidate given its involvement in telomere maintenance and prior suggestive evidence of association with melanoma/nevi [10] , [14] , [15] , as well as several other cancers. [16] , [17] , [18] PPARGC1B has previously been investigated as a skin color locus [17] and there is functional evidence for its effects on melanocytes. [18] GPRC5A (see Fig. 4a , Supplementary Fig. 15 ) has also been suggestively associated with melanoma [10] and is a known oncogene in breast and lung cancer [19] , [20] . DOCK8 deficiency predisposes to virus-related malignancy and is deleted in some cancers, but not markedly in melanoma. [21] , [22] DOCK8 regulates Cdc42 activation especially in immune effector cells—Cdc42 has been implicated in melanoma invasiveness [23] and variants in CDC42 have been previously associated with melanoma tumor thickness [24] —though our best association P value in the region of that latter gene is 3 × 10 −4 . The novel pleiotropic loci are: (a) the region around HDAC4 on chromosome 2; (b) chromosome 9q31 (two separate peaks); (c) near SYNE2 on chromosome 14; (d) in DOCK8 on chromosome 9p; and (e) near FMN1 on chromosome 15p (see Supplementary Results ). For those loci that unequivocally lie within a gene, in each case that gene is expressed in melanocytes [25] and these implicate several different pathways. The “master regulator” in melanocytogenesis [26] is MITF (microphthalmia-associated transcription factor), and we confirmed that our top candidate genes in each of the 30 regions contain MITF binding sites. [27] For example, three genes in the FMN1 region harbor MITF binding sites, viz. SCG5 , RYR3, and FMN1 themselves (enrichment P = 0.01). Furthermore, in several of these genes ( MTAP, IRF4, PLA2G6, GPRC5A , and TERC ), the most associated SNP lies within or close to the actual MITF binding sites, in some cases a rarer MITF–BRG1–SOX10–YY1 combined regulatory element (MARE) [27] (Supplementary Figs 20 – 40 ). 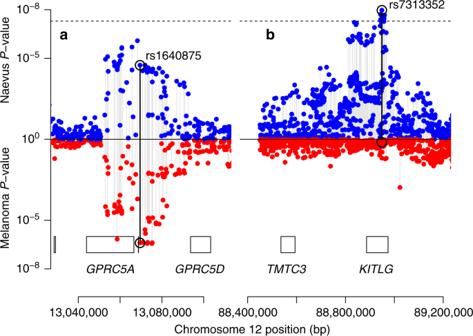Fig. 4 Plot of nevus and melanoma association testPvalues forathe region around rs1640875 inGPRC5A(chr12:12.9 Mbp) illustrating symmetrical influence on nevus count and melanoma risk; note that neither univariate peaks achieve significance alone but in combination they do (see Table2, Fig.2), andbthe region around rs7313352 inKITLG(chr12:88.6 Mbp), a “pure” nevus locus with negligible direct effect on melanoma risk Gene based tests The genes most strongly implicated in a gene-based association analysis (PASCAL) are MTAP, PLA2G6, GPR5A, ASB13 (adjacent to FAM208B ), and KITLG ( P = 2.3 × 10 −6 ); see Supplementary Table 4 ). At a suggestive level, we note FAM208B, MGC16025 (both P = 6 × 10 −6 ), and HDAC4 (1 × 10 −5 ). Among genes at a significance level of <10 −4 , we highlight LMX1B ( P = 5 × 10 −5 ), where rs7854658 gave a nevus P value of 3.3 × 10 −6 . 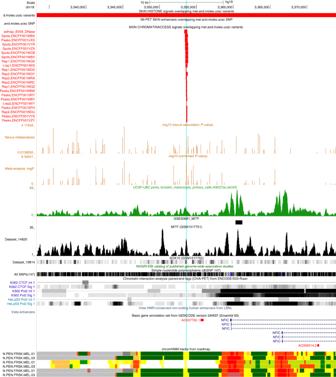Fig. 5 UCSC Genome Browser view of region nearNFIC(19p13.3). The pale blue line highlights location of rs34466956, which coincides with a narrow regulatory region as seen in in the 22 short red bars indicating open chromatin in melanocytes and skin. These align in the bottom 6 tracks with narrow yellow regions indicating results of hidden Markov models summarizing the evidence from multiple experiments for open chromatin in melanocytes. An MITF ChipSeq peak also overlies this same region (gray track, GSM1517751).NFICis expressed in melanocytes, and a second larger MITF peak overlies intron 1 in two ChipSeq experiments viz. GSE50681_MITF, see short solid black bar, and also the tall sharp gray peak below it in GSM1517751. SeeSupplementary Methodsfor details Pathway analysis Using different approaches (GWAS PRS, GWAS-PW, and REML using SNP sets; see Supplementary Table 5 ), we tested candidate pathways [28] for their overall contribution to variance in nevus number, the contribution of the telomere maintenance pathway was 0.8%. A contribution of the immune regulation/checkpoint pathway was surprisingly absent, given our knowledge that immunosuppression increases nevus count quite promptly and the recent success of CTLA4 inhibitors in the treatment of melanoma. We did see a weak signal (Combined P = 1 × 10 −7 ) for rs870191, very close to SLE-associated SNPs just upstream from MIR146A, an important immune regulator. Genetic relationships with telomere length and pigmentation In the GWAS-PW analysis combining melanoma and telomere length (TL) (see Supplementary Methods ), there was considerable locus overlap, while by contrast only TERC was detectably shared between nevus count and TL (Supplementary Fig. 41 ). Note that SNPs in OBFC1 were only significantly associated with melanoma in the phase 2 analysis of Law et al. [10] —which are not utilized in the GWAS-PW analysis—although they were suggestively associated ( P = 10 −5 ) with nevus count. In the parallel analysis with pigmentation (indexed by dark hair color), only IRF4 overlapped with nevus count (Supplementary Fig. 42 ). Again, multiple pigmentation loci acted as risk factors for melanoma (with no overlap with TL). The fact that only TERC (and OBFC1 ) are associated with nevus count, while multiple loci are associated with melanoma, is not necessarily surprising. Telomere maintenance may predispose to melanoma directly as well as via nevus count, an extension of the “divergent pathway” hypothesis for melanoma [29] . However, the link with telomere length-associated SNPs may need a bigger sample size to look at associations further. SNP heritability and genetic correlation Mixed-model twin analyses with GCTA and LDAK (see Supplementary Methods ) utilizing the Australian and British samples estimate the total heritability of nevus count to be 58% (and family environment 34%), with contributions from every chromosome and one-sixth from chromosome 9 alone (see Supplementary Table 6 ). We found that ~25% of the Australian and ~15% of British genetic variance for nevus count could be explained by a panel of 1000 SNPs covering our 32 regions. We have also performed analyses examining the overall architecture of the relationship between nevus count and melanoma risk using bivariate LD score regression analysis and estimated r g = 0.69 ( SE = 0.16) (see Supplementary Results ). Alleles which increase nevus number proportionately increase the risk of melanoma ( Supplementary Results , Supplementary Figs 43 , 44 ) with KITLG, the interesting exception is that the nevus-associated variants did not predict melanoma risk (see Fig. 5b ), rather, predisposing to other cancers (e.g., testicular germ cell). It has been long suggested that carrying out genetic analyses using multiple correlated phenotypes will increase power to detect trait loci in such a way as to justify the statistical complications. Since number of cutaneous nevus is strongly correlated with melanoma risk, and known nevus loci were associated with CM, it seemed likely that this would be a fruitful approach. We have highlighted eight novel loci, including the genes HDAC4, SYNE2 , and most notably GPRC5A , where quite large samples of melanoma cases or nevus count were not sufficiently powerful to reach formal genome-wide significance in univariate analyses, but the combined evidence is conclusive. Given that lighter skin color is also associated with both these phenotypes, we would expect a strong contribution from pigmentation pathway genes. Among those novel pleiotropic loci implicated in nevus count, CYP1B1 and PPARGC1B both appear in a recent skin pigmentation meta-analysis [30] as harboring variants lightening skin color. The SNPs in the chromosome 7p21.1 region near AHR and AGR3 previously associated with CM also appear to be associated with skin color in that study. In our analysis, the signal for nevus count from that interval (best P = 3 × 10 −4 ) was half as strong as that for CM, and the GWAS-PW analysis support was equal for the hypotheses of a pure CM locus and a pleiotropic locus (region PPAa = 0.494, PPAc = 0.485). In passing, the peak SNPs lie within a long noncoding RNA gene ( TCONS_I2_00025688 ) that is expressed in melanocytes, so this is a potential candidate for both skin color and CM. In the case of KITLG , the variant most strongly associated with pigmentation (fair hair), rs12821256, modifies a distant enhancer, and was associated neither with melanoma or nevus count in our study (see Supplementary Results ). We observe a similar pattern (association P nevus = 0.4, P CM = 0.8) for the strongest associated variant for skin color from the skin color meta-analysis, rs11104947. [30] By contrast, HDAC4 and DOCK8 are in pathways that have not been implicated as important to nevogenesis or melanoma pathogenesis. HDAC4 is involved in transcriptional regulation in many tissues, while DOCK8 acts to regulate signal transduction, most notably in immune effector cells (see Supplementary Results ). The association peak for HDAC4 is quite wide (~80 kbp), and overlaps with the multi-tissue GTEx eQTL peak for this gene. [31] The best overlapping SNP was rs115253975, with a combined nevus-CM P -value of 4 × 10 −9 and fibroblast HDAC4 eQTL P -value of 2 × 10 −5 . The peak nevus-CMM DOCK8 SNP, rs600951, is a cis-eQTL in two (non-cutaneous) tissues, and the peak around it contains several eQTL SNPs detected in the GTEx skin samples. These eQTL SNPs would be potential causal candidates. Both SYNE2 (encoding nesprin-2) and FMN1 (formin-1) are involved in nuclear envelope and cytoskeleton function, and through this in regulating as well as facilitating numerous biological pathways. Both, for example, are involved in directed cell migration. The nesprin and formin families have been implicated in efficient repair of double strand DNA breaks, so this might point to a mechanism for an association with nevi and CM (see Supplementary Results ). We did see heterogeneity between studies in strength of SNP association with nevus count or melanoma for four loci, most extremely for IRF4 (Supplementary Fig. 10 ). Meta-regression analysis suggested this is partly due to interactions with age in the case of IRF4 (Supplementary Table 1 )—different nevus subtypes are known to predominate at different ages, with the dermoscopic globular type most common before age 20. [32] We suspect sun exposure another important interacting covariate, given large differences in total nevus count by latitude. [33] , [34] Epidemiologically, the etiology of melanoma has been divided [35] into a chronic sun-exposure pathway and a nevus pathway, where intermittent sun exposure is sufficient to increase risk. At a genetic level, pigmentation genes such as MC1R contribute only via the former pathway (though this can include effects on DNA repair [36] ), others such as MTAP via the latter, while yet others such as IRF4 seem to act via both routes [13] . We interpret our results as consistent with the hypothesis that nevus number is the intermediate phenotype in a causative chain to melanoma originating in all these biologically heterogeneous nevus pathways. However, we acknowledge that there may also be some genes where there is a direct causal pathway to both phenotypes. We carried out a meta-analysis of 11 sizeable GWAS of total nevus count in populations from Australia, Netherlands, Britain, and the United States, subsets of which have been reported on previously [5] , [6] , [8] , and then combined these results with those from a recently published meta-analysis of melanoma GWAS [10] to increase power to detect pleiotropic genes. While nevus counts or density assessments are available for melanoma cases from a number of studies, in the meta-analysis of nevus count we included only samples of healthy individuals without melanoma, all of European ancestry (for more details, see Supplementary Methods ). Nevus phenotyping The assessment of nevus counts varies considerably between the 11 studies in four respects (see Table 1 ): (a) nevus counts vs. density ratings; (b) whole body vs. only certain body parts; (c) all moles (> 0 mm diameter) or only moles >2 mm, or 3 mm, or 5 mm; and (d) count by trained observer or self-count by study participant. These differences could contribute statistical heterogeneity into our analyses, so we have done considerable preliminary work to convince ourselves that all assessments are measuring the same biological dimension of “moliness” (see Supplementary Fig. 3 ). A pragmatic test of this is the relative contribution of each study to the detection of the known loci of large effect, which is evident from the forest plots (Supplementary Figs 5 – 19 ). Statistical methods Given this, we combined results from each study as regression coefficients and associated standard errors in standard fixed and random effects meta-analyses using the METAL [37] and METASOFT [38] programs. Manhattan and Q–Q plots for the nevus GWAS meta-analysis (GWASMA) are shown in Supplementary Fig. 45 and for each of the contributing studies in Supplementary Figs 46 – 55 . We combined the results from the nevus meta-analysis above with results from stage 1 of a recently published meta-analysis of CM [10] . Stage 1 of the CM study consisted of 11 GWAS data sets totaling 12,874 cases and 23,203 controls from Europe, Australia, and the United States; this stage included all six published CM GWAS and five unpublished ones. We do not utilize the results of stage 2 of that study, where a further 3116 CM cases and 3206 controls from three additional data sets were genotyped for the most significantly associated SNP from each region, reaching P < 10 −6 in stage 1. As a result, certain melanoma association peaks are not genome-wide significant in their own right in the present bivariate analyses. Further details of these studies can be found in the Supplementary Note to Law et al. [10] . The combination of the nevus and melanoma results was performed using the Fisher method. A Manhattan plot for the combined nevus GWASMA plus melanoma GWASMA is shown in Supplementary Fig. 4 . For more details of statistical methods, see Supplementary Methods .